Forests fuel fish growth in freshwater deltas Aquatic ecosystems are fuelled by biogeochemical inputs from surrounding lands and within-lake primary production. Disturbances that change these inputs may affect how aquatic ecosystems function and deliver services vital to humans. Here we test, using a forest cover gradient across eight separate catchments, whether disturbances that remove terrestrial biomass lower organic matter inputs into freshwater lakes, thereby reducing food web productivity. We focus on deltas formed at the stream-lake interface where terrestrial-derived particulate material is deposited. We find that organic matter export increases from more forested catchments, enhancing bacterial biomass. This transfers energy upwards through communities of heavier zooplankton, leading to a fourfold increase in weights of planktivorous young-of-the-year fish. At least 34% of fish biomass is supported by terrestrial primary production, increasing to 66% with greater forest cover. Habitat tracers confirm fish were closely associated with individual catchments, demonstrating that watershed protection and restoration increase biomass in critical life-stages of fish. Conserving the world’s freshwater ecosystems requires protecting both water bodies and the terrestrial habitats surrounding them. This is because biological, chemical and physical processes in water depend on organic matter (OM) derived from terrestrial vegetation and soils. Between 20 and 85% of secondary production in different freshwater ecosystems is derived from terrestrial OM [1] , [2] and these inputs also influence water quality and thermal structure [3] . Changes in OM exports from terrestrial catchments, associated with factors such as climate change, industrial activities and land-use change [4] , [5] , might therefore have far-reaching consequences for managing freshwater ecosystems and the vital ecological services they provide. Fish stocks (that is, biomass) are one service provided by aquatic ecosystems that vary with the delivery of terrestrial OM. However, the direction of their response will depend on whether existing aquatic productivity is reduced as terrestrial OM flows into lakes [6] . In general, once exported from land, some OM is dissolved in water and mobilized upwards through food webs by bacterial assimilation and growth [1] . Large particulate OM can also be ingested directly by consumers and metabolized by bacteria through decomposition [7] , [8] , [9] . Fish consequently intake OM produced outside (allochthonous) rather than within (autochthonous) lake boundaries by consuming benthic macroinvertebrates and zooplankton supported by OM originally derived from land. In north temperate regions, where most lakes are relatively small (<1 km 2 ) and increasingly less productive [10] , [11] , allochthonous subsidies can account for most of the food resources used by fish [2] , [8] , [12] . This suggests that as terrestrial inputs of OM increase, so too might bacterial production, macroinvertebrate and zooplankton biomass, and ultimately fish yields [1] , [6] , [8] , [13] . However, declines in secondary production may arise if terrestrial inputs are sufficiently large and/or coloured so as to shade aquatic primary production [6] , [14] . Food quality also factors into the debate. A central argument against large allochthonous support of fish populations has been that terrestrial OM lacks high-quality nutrients, such as essential fatty acids, needed to support zooplankton and other consumers [15] , [16] . Reductions in water clarity can lower the amount of fatty acids (FA) that consumers obtain from their food by dampening primary production and shifting algal communities to less nutritionally rich species [17] . Consumers may consequently have to ingest more food to maintain their growth, reducing the benefit of elevated OM [18] . However, OM may continue to be beneficial in at least two circumstances. First, both food quantity and quality can increase in nutrient-limited systems with high light penetration if nitrogen and phosphorus associated with terrestrial OM stimulate primary production [19] . Second, terrestrial OM is a source of n-6 FA for invertebrates in littoral zones, transferring FA up food webs [20] and potentially minimizing the impact of reduced primary production from shading. The boreal ecozone contains ≥60% of the world’s surface freshwater, but little is known about how aquatic ecosystem services will change there as terrestrial OM export is altered by anthropogenic activities [21] . By using a gradient of forest cover as a space-for-time substitution, we tested whether disturbances that removed terrestrial biomass lowered OM inputs into freshwater lakes and reduced the productivity of aquatic food webs. Previous work has estimated the relative contribution of terrestrial OM towards different trophic levels [22] , [23] , [24] , but not how changes to land cover affect aquatic biomass in the boreal. Most food webs in boreal lakes extensively use terrestrially produced OM because they are nutrient poor [25] , [26] , and our aim was to quantify the watershed characteristics that modify this dependency. We focused on eight near-shore sites receiving inputs from separate sub-catchments within a 275 ha watershed in Ontario, Canada. Our system provided a unique opportunity to test the importance of terrestrial OM subsidies in supporting aquatic biota because of strong gradients in vegetation and soil development, but not mean lake water chemistry, among sites. Focusing on the stream-lake interface had the added benefit of capturing the effects of terrestrial subsidies within small areas of biological activity, which are important to the life stages of many organisms. Our approach was to test whether the biomass of fish increases with forest cover and terrestrial OM inputs of each sub-catchment, and then quantify the extent to which they consist of allochthonous OM using stable isotope analyses (SIA). We focused on the widely distributed yellow perch ( Perca flavescens , hereafter ‘perch’), an important sport and commercial species throughout North America. Young-of-the-year (YOY) perch are particularly suited for reflecting near-shore habitats because they colonize different sites in a lake from a common pool of interspersed juveniles [27] . Larvae hatch en mass in response to favourable temperatures and immediately move to the pelagic zone where they are mixed by water currents. Once individuals are large enough to swim against water currents ( ca . 2 weeks in small lakes), they disperse into littoral sites [27] , seeking habitat in which to escape predators and feed as planktivores [28] . It is during this period that size differences emerge [29] . We predicted that greater forest cover exports more OM from land as particulate organic carbon (POC), elevating dissolved organic carbon (DOC) and eventually biomass of bacteria, zooplankton and YOY perch. Using generalized linear models, we tested whether each of these responses, measured at the site level or averaged within sites where replication was possible, increased with the quantity of OM in the first trophic level directly underneath in the lake food web. More generally, we ascribe differences in the productivity of sites to varying amounts of energy flowing upwards through similar food webs and term this process a ‘trophic upsurge’. Our intention is to contrast the paradigm of trophic cascades, which predicts differences in productivity, and ultimately biomass stocks, arise from variation in food web structure rather than energy supplies [30] . In addition to food quantity, we accounted for the variation in biomass of each trophic level explained independently of the upsurge hypothesis by food quality, such as essential FA content for YOY perch. Overall, we provide direct evidence that forest cover can promote the biomass of fish in the boreal lakes that hold most of the world’s freshwater. Trophic upsurge We found strong support for the trophic upsurge hypothesis. 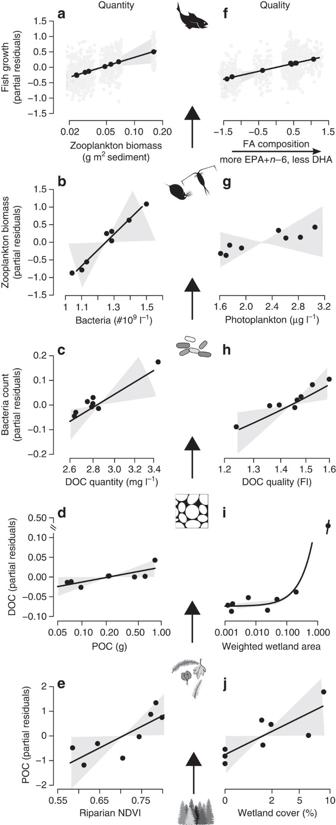Figure 1: Evidence for the trophic upsurge hypothesis. Biomass and concentrations of (a) YOY fish, (b) zooplankton (relativized per area of lake sampled), (c) bacteria, (d) DOC and (e) POC increase in each site (n=8) with the amount of OM in subordinate trophic levels. (f–j) Influence of OM quality, with strongest predictor plotted (seeTable 1). Lines are mean model fit±95% CIs in shaded polygons. Points ina,fare residuals for site-level means, although we considered individual variation shown in grey (n=800). No relationship plotted ing, because slope overlapped zero. Raw data for all response variables presented as predictors alongxaxes, except for fish weights that are shown inSupplementary Table 2. All parameter estimates are reported inSupplementary Table 3. By controlling for explanatory variables, such as habitat condition and food quality, we assessed the power of food quantity to predict the amount of OM at different trophic levels across our eight study sites using generalized linear models ( Table 1 ). As expected, the resulting partial residuals suggested that terrestrial OM export percolated upwards through the aquatic food web ( Fig. 1a–e ). Allochthonous POC trapped in deltas increased with riparian forest cover surrounding each site (95% credible interval (CI) for effect: 0.03–1.44), and was associated with greater DOC concentrations averaged across the period of POC sampling (95% CI for effects non-overlapping zero: 0.01–0.03). The presence of wetlands at one site also strongly promoted DOC, presumably through a terrestrial POC–DOC pathway consistent with the upsurge hypothesis ( Fig. 1 ). As DOC increased in each site delta, so too did bacterial densities (95% CI: 0.02–0.14). Greater densities of bacteria were then associated with increased zooplankton biomass at the site-level (95% CI: 0.10–1.32) and more zooplankton was associated with greater mean fresh weights of perch at each site (95% CI: 0.07–0.49). Weights were uninfluenced by perch abundance, independently estimated from gillnet surveys (95% CI: −0.14–0.07; Supplementary Methods ); hence, differences in fish size were not due simply to variation in the numbers of individuals consuming resources at each site. Table 1 Responses of trophic levels and organic carbon export to the quantity and quality of their organic matter inputs. Full size table Figure 1: Evidence for the trophic upsurge hypothesis. Biomass and concentrations of ( a ) YOY fish, ( b ) zooplankton (relativized per area of lake sampled), ( c ) bacteria, ( d ) DOC and ( e ) POC increase in each site ( n =8) with the amount of OM in subordinate trophic levels. ( f – j ) Influence of OM quality, with strongest predictor plotted (see Table 1 ). Lines are mean model fit±95% CIs in shaded polygons. Points in a , f are residuals for site-level means, although we considered individual variation shown in grey ( n =800). No relationship plotted in g , because slope overlapped zero. 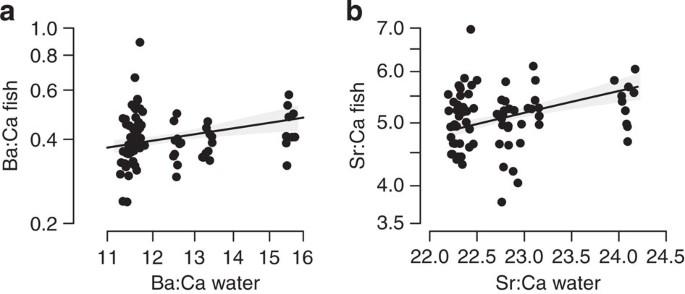Figure 2: Molar ratios in fish increase with those in water at each site. We focused on ratios of (a) Ba:Ca and (b) Sr:Ca. Solid line is model fitted at mean fish body mass and level of wetland influence, with shading denoting 95% CIs. Values in thexaxis were jittered for clarity (n=77; 3 fish could not be analysed). Parameter estimates reported inSupplementary Table 4. Raw data for all response variables presented as predictors along x axes, except for fish weights that are shown in Supplementary Table 2 . 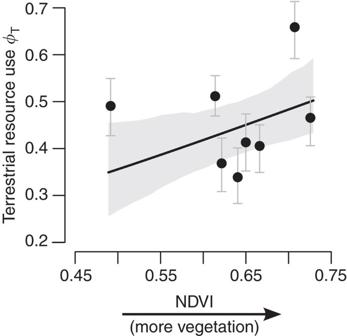Figure 3:Terrestrial resource use (φT) by YOY perch increases with vegetation cover in terrestrial catchments. Symbols are meanφT±95% CIs estimated within each site from a three-isotope mixing model (n=8). Solid line is model fitted at median value of wetland cover and catchment size with shaded area denoting 95% CI. All parameter estimates are reported inSupplementary Table 3. All parameter estimates are reported in Supplementary Table 3 . Full size image Trace metal signatures of perch helped to validate our experimental design. Perch populations in each site had distinct metal signatures ( Supplementary Fig. 1 ), with individual fish reflecting the water chemistry from their site of capture ( Fig. 2 ). Thus, YOY perch showed close affinity to the littoral habitats from which they were captured, demonstrating that they were products of their local catchments between the larval and juvenile growth periods. Figure 2: Molar ratios in fish increase with those in water at each site. We focused on ratios of ( a ) Ba:Ca and ( b ) Sr:Ca. Solid line is model fitted at mean fish body mass and level of wetland influence, with shading denoting 95% CIs. Values in the x axis were jittered for clarity ( n =77; 3 fish could not be analysed). Parameter estimates reported in Supplementary Table 4 . Full size image Increasing food quality generally promoted the biomass of trophic levels, but it did not explain more of the variation in the weights of YOY perch than food quantity ( Table 1 ). Weights of fish increased with the proportion of high-quality FA in zooplankton communities at each site (95% CI: 0.14–0.49), and this was not more important than the positive effect of zooplankton biomass (evident by overlapping CIs in Table 1 ). We summarized FA composition with a single index that increased with eicosapentaenoic acid (EPA, 20:5n-3; 95% CI: 0.42–1.67) and n-6 FA (95% CI: 0.52–1.78), dominated by linoleic acid (18:2n-6) and arachidonic acid (20:4n-6) found in larger invertebrates [31] . Increasing values of this index were, however, associated with less docosahexaenoic acid (DHA, 22:6n-3) at each site (95% CI: −1.71 to −0.36). This is because different zooplankton communities accumulate DHA than those that accumulate EPA, and so the two FA are strongly inversely correlated (Spearman’s rank correlation: ρ =−0.88, P =0.007). Specifically, DHA declined where we found relatively more Cladocera than Copepoda species, while the relative amount of EPA increased ( ρ =−0.76, P =0.037 and ρ =0.81, P =0.022, respectively; Supplementary Fig. 2 ). Individual Cladocera also had lower mass fractions of DHA than co-occurring Copepoda in our sites ( Supplementary Table 1 ). Additional measures of habitat quality also explained variation in the biomass of trophic levels ( Table 1 ). For example, bacterial densities increased with less structurally complex OM, estimated with the fluorescence index, and the delivery of OM to the lake-stream interface increased with wetland coverage, measured from aerial photographs ( Table 1 ). Critically, none of these effects were stronger than those associated with the quantity of OM in different trophic levels (that is, absolute effects overlapping or less than those of quantity in Table 1 ). The sole exception was DOC ( Table 1 ), which was strongly influenced by one site with a disproportionately large wetland ( Fig. 1i ). Other models that might have potentially explained differences in biomass stocks, such as trophic cascades or variation in fish hatching dates, were also poorly supported when compared with our upsurge hypothesis ( Supplementary Note 1 and Supplementary Table 2 ). Terrestrial resource use by fish Both aquatic production and terrestrial inputs were important resources for fish as estimated with a three-isotope mixing model [23] . Between 34 and 66% of the isotopic signature (δ 2 H, δ 13 C and δ 15 N) of YOY perch was estimated to be derived from terrestrial resources, with an increasing reliance on these as both the density of forest vegetation and wetland cover increased in the local catchment (95% CIs overlapping: 0.15–0.58 and 0.11–0.42, respectively; Fig. 3 ). The positive effect of vegetation density also increased with wetland cover (95% CI for interaction: 0.26–0.69), supporting the idea that sites with a greater potential for waterlogging provided additional OM during periods of high runoff [32] . However, terrestrial support was lower as catchments increased in size (95% CI: −0.53 to −0.12), suggesting that larger sites are more likely to trap OM within microsites because material traverses greater distances during export [33] , [34] . Figure 3: Terrestrial resource use ( φ T ) by YOY perch increases with vegetation cover in terrestrial catchments. Symbols are mean φ T ±95% CIs estimated within each site from a three-isotope mixing model ( n =8). Solid line is model fitted at median value of wetland cover and catchment size with shaded area denoting 95% CI. All parameter estimates are reported in Supplementary Table 3 . Full size image Despite the terrestrial influence, within-lake support for YOY perch was greater in five of the eight sites when estimating the relative use of different resources. This does not diminish the relative importance of terrestrial resources, which we found to have overlapping effects with autochthonous resources when predicting fish growth ( Table 1 ), as the extent to which resources are used can differ from their importance. Littoral resources (i.e., vertically migrating zooplankton in the near-shore photic zone) accounted for between 32 and 59% of the isotopic signature of fish, except at one site where they were only 6% of the signature and benthic support was much higher ( Supplementary Table 3 and Supplementary Fig. 3 ). Overall, our model closely predicted site-level isotopic ratios ( R 2 for posterior means=0.47–0.99; Bayesian R 2 incorporating residual uncertainty=0.45–0.58; Supplementary Fig. 4 ), and stable isotope ratios of littoral zooplankton and benthic periphyton were distinct from those of leaf litter, allowing us to separate terrestrial resources from autochthonous sources ( Supplementary Fig. 5 ). Our study shows how the biomass of YOY perch is shaped by land use and this has important generalities for the production of fish stocks. We found that the biomass of fish increased with the amount of OM transferred upwards through the aquatic food web, and the export of OM from land increased as more of the near-shore area was forested and covered by wetlands. To our knowledge, this is the first time this has been demonstrated across landscape-level gradients of vegetation cover, extending findings within pelagic mesocosms [13] , [35] . Our results also have consequences beyond YOY fish because recruitment into adult fish stocks and subsequent population dynamics are strongly size-dependent in perch [28] and other species [36] . Therefore, terrestrial subsidies should continue to be mobilized upwards through aquatic food webs from adult forage species to their predators [8] , [24] . Although fish increasingly relied on these resources as more of the land was forested, reaching 66% terrestrial support in the most vegetated sites, measuring the use of resources with stable isotopes is different from estimating their relative importance [23] , which we accomplished by modelling the trophic upsurge hypothesis. Models of the upsurge hypothesis discounted a simple substitution of terrestrial for autochthonous resources with increasing forest cover [23] , as fish equally relied on both essential FA produced by phytoplankton, such as EPA, and the quantity of zooplankton biomass available at each site, which was a product of terrestrial OM ( Table 1 ). Rather, we suggest that the greater absolute export of particulate OM from more forested catchments provides an additional food source that subsidizes fish growth, and these subsidies are increasingly important as forest and wetland cover increase. Most of this subsidy will come from particulate OM, as it is deposited directly into stream mouths, while dissolved OM delivered by streams will remain suspended and move to pelagic zones, likely to be contributing little to near-shore habitats [37] . Importantly, the resulting differences in fish size associated with these subsidies are sufficiently large to alter overwinter survival, predation risk and competitive interactions [28] . In no way does this diminish the influence of autochthonous resources, which are used at high amounts according to SIA, although they are not the sole drivers of secondary production as shown with statistical models of the upsurge hypothesis. Inputs of terrestrial OM increased allochthonous support of lake food webs, suggesting that they diluted the relative contribution of autochthonous production to secondary production, perhaps by reducing water clarity. Although OM inputs can elevate nitrogen (N) and phosphorus (P) available for phytoplankton growth through photolytic release [38] and stimulating bacterial decomposition [39] , [40] , the benthic algae that dominate primary production in littoral zones of north temperate lakes [41] are more limited by light than nutrients [14] . In our study, DOC concentrations, which increased from terrestrial OM subsidies ( Table 1 ), were positively associated with water colour ( ρ =0.52, P <0.001, n= 64) and more coloured water reduces light penetration [42] . Consequently, relative increases in the summed abundance of algal groups between measurements recorded every 2 to 5 days were smaller as water became relatively darker ( ρ =−0.30, P =0.029); despite that DOC was positively associated with total P and Kjeldahl N ( ρ =0.28, P =0.028 and ρ =0.25, P =0.046, respectively). This may help explain why the relative contribution of autochthonous sources towards fish production declined in sites where forest cover and hence DOC were consistently higher. Although increasing terrestrial OM may contribute proportionately more towards aquatic food webs and promote their productivity, these effects may reach a threshold at very high concentrations [6] . At high OM concentrations, shading of photosynthesis, and the poor substrate availability and acid-neutralizing capacity of humic compounds, can limit basal food production and reduce fish biomass [6] , [14] . Terrestrial support will also not continue to increase with forest cover if shading limits food quality, such as phytoplankton taxa that produce the FA essential to fish growth. However, this was not evident here. Overlapping CIs in our models showed EPA produced by phytoplankton was as important for fish as n-6 FA, which can be derived from processing of terrestrial OM by benthic macroinvertebrates in littoral zones [20] . Our work helps to reconcile an important debate: whether allochthonous OM can support a high proportion of the production within higher trophic levels given the nutritional requirements of consumers for autochthonous resources [8] , [13] , [15] , [16] , [22] , [23] . We achieved this by demonstrating that terrestrial OM subsidizes rather than replaces autochthonous resources and the strength of this subsidy depends on the characteristics of surrounding catchments, which have varied among past studies. Two key results support these assertions. First, we estimated the relative importance of allochthonous and autochthonous resources for increasing the biomass of different trophic levels and found that these effects can overlap. For example, weights of YOY fish increased with both zooplankton biomass, stimulated by terrestrial OM, and FA produced within lakes. Second, we measured support of consumers by allochthonous resources with stable isotopes and showed that it was correlated positively with forest and wetland cover, only reaching higher values (i.e. 66%) in more vegetated sites. These sites export the most OM and are typical of those in the boreal ecozone [21] , [43] , where the majority of the world’s freshwater is found [21] . Our results, in combination with other studies, thereby suggest that terrestrial support of aquatic consumers will be highest in nutrient-poor systems, where allochthonous OM inputs are much greater than algal production [2] , [8] , [15] , [23] . Previous disagreements over the importance of terrestrial support may have arisen because lakes such as ours, and those in Scandinavia and Wisconsin (for example, refs 7 , 8 , 44 ), are surrounded by different types of vegetation than those in the western United States, where allochthonous support is considerably lower [16] , [45] . This may have two consequences. First, riparian plant communities dominated by deciduous trees in the western United States will export relatively lower quantities of particulate and dissolved OM than communities surrounded by slower decomposing coniferous species [46] , [47] , which occur throughout the boreal. Land use around some western US lakes, i.e. urbanization, may also be reducing terrestrial subsidies [48] . Second, deciduous trees export OM that has a different structural complexity and hence availability to bacterial communities [49] , [50] . Wetlands that are widespread in boreal regions also produce high amounts of humic substances [49] , which reduce autochthonous production [6] , [14] . Overall, such differences in the quantity and quality of OM exported by land may help explain variation in terrestrial support of aquatic secondary consumers. For example, DOC can contribute little to lake food webs at low levels, such as that found in the western United States [46] , but increasingly benefit secondary consumers at the higher concentrations found in boreal regions [6] . These benefits will accumulate until they are outweighed by larger reductions in the quantity and quality of autochthonous resources associated with elevated DOC [6] , [14] . Clearly, our results show how the debate over allochthony must be placed within the context of surrounding watershed characteristics and management practices [34] . A critical question emerging from our study is whether trophic levels are responding to bottom-up drivers or whether the drivers are themselves responding to top-down control. Obviously, our food web data will reflect the reciprocal influences of both top-down and bottom-up forces, but evidence from testing our trophic upsurge hypothesis suggests that the latter is more important in our system. For example, we found no effect of zooplankton biomass on bacterial densities and zooplankton themselves were not reduced by fish more than the extent to which they increased with bacteria ( Table 1 and Supplementary Note 1 ). Experiments are now needed to measure how the effects of trophic cascades on upsurges vary with biological, chemical and physical properties of lakes and their surrounding catchments [34] . Responses of aquatic ecosystems under different environmental conditions can also be coupled to terrestrial dynamics using watershed- and regional-level simulation models (for example, refs 51 , 52 ). Such models can help to predict the effects of global change on ecosystem services, such as fish stocks, and can aid restoration of degraded landscapes by identifying impediments to biological recovery. Consumption of fish is vital for human well-being; thus, there is a need to predict how land-use change will alter the delivery of this important ecosystem service. Fish supply nearly 7% of global protein consumption, as estimated from country-level trade statistics and standardized nutritional tables [53] , and are by far the primary source of dietary n-3 FA that reduce risk of diseases in humans [54] . Our results now suggest that anthropogenic disturbances, such as fire and logging, which are increasingly removing large amounts of plant biomass from boreal forests [21] , should reduce export of terrestrial OM and subsequently the biomass of aquatic food webs, until vegetation recovers to a pre-disturbance state (for example, ref. 47 ). Terrestrial OM and nutrients are, however, exported at elevated rates immediately after disturbance (≤3 years) because removal of vegetation: (i) raises water tables, through lowering evapotranspiration, (ii) stimulates microbial activity, by increasing soil moisture and temperature, and (iii) supplies coarse debris [55] . Therefore, the conservation of productive fisheries in small boreal lakes must extend up-shore into riparian areas and coordinate with land planning through much broader watershed-level management. Our study region (Sudbury, Canada) offers a unique example of such cooperation. Intensive restoration of acid- and metal-damaged lakes over the past 40 years has focused on surrounding catchments by neutralizing acidified soils, planting millions of trees and herbaceous plants, and protecting wetlands [56] . We now show that such efforts deliver measurable benefits to aquatic ecosystem services and human food supplies. Study area We studied 8 of 16 sub-catchments that varied most widely in forest cover around Daisy Lake, Sudbury, Ontario (46°27′N, 80°52′W; lake area=36 ha; maximum depth=14 m). The watershed has a distinct gradient of terrestrial recovery from historical acid and metal contamination, increasing with distance from a nickel smelter that was closed in 1972 and located 3.5 km to the northeast ( Supplementary Fig. 6 ). Given its proximity to the smelter, the lake was acidic (pH<5.0) and metal contaminated from the 1940s to the 1980s, but has since recovered to a pH of near 7 due to regional pollution controls and the absence of other large-scale disturbances [37] . Lake water pH does not vary among our eight study sites, as 95% CIs overlapped for the mean pH predicted in each site from semi-weekly samples collected between May–July 2012. Barren and eroded substrates around the lake are also slowly being recolonized by trees and shrubs, primarily paper birch ( Betula papyrifera ) and trembling aspen ( Populus tremuloides ), particularly where soil layers remain intact. Eight species of fish have re-colonized since 2000 from a connected lake. We focused all our sampling over a depth of 0.25–0.75 m outwards from the interface between each sub-catchment stream and the lake. The eight sub-catchments that we studied function relatively independently because they have unique soils and geomorphologies. Thus, they provide us with multiple units of study despite being located within the same watershed. Vegetation density in each sub-catchment was estimated using the normalized difference vegetation index (NDVI), a widely used indicator of photosynthetic absorption that is derived from remote sensing imagery (see Supplementary Methods ). High values of NDVI distinguish forest from herbaceous vegetation and barren surfaces. Quantity of organic OM at different trophic levels We sampled OM, bacteria, phytoplankton and zooplankton at each site during the summer of 2012, immediately before collecting YOY yellow perch. POC and DOC : We measured the quantity of POC and DOC in each site. We installed eight 50-ml polypropylene centrifuge tubes (3 cm diameter) at a depth of ca . 0.5 m in the centre of each site on 22 May 2012 to collect particulate material (after ref. 37 ). Tubes were extracted on 24 June 2012, and contents rinsed through a 250-μm mesh. The filtrate was then homogenized and vacuum-filtered onto Whatman glass microfibre filters (GE Healthcare Bio-Sciences Corp., Piscataway, NJ). This retained material 1.5–250 μm in size, capturing the range of OM used by consumers [57] , [58] . Material on the filters was then oven dried at 60 °C and combusted at 500 °C, whereby mass loss after combustion served as our measure of POC quantity. Two water samples were also collected per week from the mid-water column ( ca . 0.5 m) in the centre of each site and immediately filtered through an 80-μm mesh. Samples were measured for DOC using automated colorimetry, and should capture the range of molecules <1.5 μm in size [59] . Bacteria : We measured bacteria from one water sample per week collected concurrently for DOC. In the lab, 0.5 ml subsamples of water were filtered undiluted through a 0.2-μm black polycarbonate membrane and stained with 25 μl 4′,6-diamidino-2-phenylindole. Immediately before exposure of each sample to fluorescence, we added a drop of SlowFade Antifade reagent to reduce photobleaching (Life Technologies Corporation, Carlsbad, CA). We then counted bacterial cells in ten random fields from each subsample beneath an epifluorescent microscope to derive bacterial densities. Phytoplankton : We measured phytoplankton biomass in the water samples collected concurrently for DOC using a chlorophyll fluorometer (bbeMoldaenke, Kiel-Kronshagen, Germany) as the summed concentrations (μg l −1 ) of diatoms and chrysophytes (Bacillariophyceae), green algae (Chlorophyceae), cyanobacteria (Cyanophyceae) and cryptophytes (Cryptophyceae). By measuring fluorescence excitation at 370, 470, 525, 570, 590 and 610 nm, concentrations of different taxonomic classes can be estimated from their specific chlorophyll absorption spectra. Biomass estimated with this approach has been validated with traditional methods, such as HPLC, chlorophyll extraction and physical counts of algal cells [60] , and increased with chlorophyll a concentrations in our samples measured using spectrophotometry ( ρ =0.32, P =0.011, n= 64). Importantly, fluorescence measurements were not confounded by variation in true water colour measured using colorimetry ( ρ =0.02, P =0.865). Zooplankton : We collected free-floating littoral zooplankton nightly on 4 and 5 July 2012 in each site. Night-time funnel traps collect complementary species to daytime hauls in littoral zones, as well as species that are inactive during the day [61] . Animals were captured with nine 500-ml vertically deployed funnel traps positioned at a distance of ≥1 m from each other. We collected traps the morning after deployment and immediately filtered samples through a 1,250-μm mesh. By collecting animals ≥1,250 μm in size, we focused on the range of zooplankton likely to be consumed by YOY perch [62] , [63] . Retained material was washed into a vial with Milli-Q water and refrigerated for ca . 4 h to allow for digestion, assimilation and/or gut evacuation [64] . Samples were then live-sorted into pure zooplankton and evenly divided into two subsamples using a Folsom plankton splitter. The first subsample was flash frozen on dry ice until used for measuring biomass and FA (described in Supplementary Materials ), while the second was freeze-dried and ground into a fine powder for SIA. To have sufficient mass for analyses, we pooled samples for FA ( n= 3 per site) and from the same trap between nights where necessary for SIA ( n= 3–9 per site). Zooplankton were sampled only on the two dates, because their isotopic and FA signatures are likely to have been relatively stable across the few weeks during which fish would have been large enough to be planktivorous. Signatures mainly vary across larger temporal scales, such as seasonally between winter and summer [65] . Fish : We captured YOY perch at each site on 5 July 2012 using a purse seine (mesh size=0.3 cm; depth=1.2 m; length=15.2 m). Caught individuals were euthanized and immediately refrigerated. We recorded the mass of 100 randomly selected individuals from each site. Fifteen individuals per site were freeze-dried and ground into a fine powder for SIA (after ref. 7 ). Other studies sample muscle tissue for SIA (for example, ref. 23 ). However, this is often intended as a proxy for whole-body isotope signatures, and thus may be inappropriate in small fish (<90 mm), where whole-body samples can be directly measured more accurately and sufficient mass for analyses can be obtained without pooling individuals into composites [66] . Stable isotope ratios We collected leaf litter and periphyton at each site and analysed these with zooplankton and fish (described above) for δ 2 H, δ 13 C and δ 15 N on isotope-ratio mass or cavity-ring-down laser spectrometers at the Colorado Plateau Stable Isotope Laboratory, University of Northern Arizona. Terrestrial signature : We sampled plant litter in June 2012 to measure allochthonous sources of OM. Within each sub-catchment, we collected all loose litter >850 μm in size from the soil surface within 0.25 m 2 plots. Plots were located at random bearings at a distance of 1, 3, 5, 7 and 9 m from the mouth of the riparian drainage streams, as most leaf litter exported into lakes is derived from within this distance of streams [67] . Litter was oven-dried at 60 °C and finely ground into a homogenous mixture. We calculated spatially weighted averages for isotopic ratios from the different distances within each sub-catchment. Both vegetation and soils did not vary with distance from the stream mouth; hence, the 9-m sampling area probably captures OM sources at similar positions from across the much larger catchments. Approximately 75% of basal area measured across seven of our eight study catchments in 2008 was dominated by Betula papyrifera [37] , and the amount of birch basal area did not vary with distance within 100 m of the stream mouth ( ρ =−0.05, P =0.596). Partly, this may have arisen because both per cent canopy cover and the depth of the humic layer did not change as we moved upwards into catchments ( ρ =−0.03, P =0.771 and ρ =−0.15, P =0.111, respectively). Periphyton : We sampled stable isotope ratios of periphyton at each site to measure within-lake support of fish. We anchored three 16-cm diameter unglazed clay discs 0.10 m above the lakebed in the centre of the channel emerging into the lake from each sub-catchment stream. Discs remained positioned from 22 May to 24 June 2012 to allow periphyton to accumulate. This approach allows benthic algae to be isolated much more readily than if periphyton was collected from natural substrates [68] . On removal, discs were scraped of material and samples freeze dried. Periphyton, which is a mixture of bacteria, phytoplankton and detritus, may be a more robust indicator of within-lake OM production because it integrates temporal variability in bacteria and phytoplankton. Many studies in fact sample mixtures of these microorganisms as periphyton, because isolating pure phytoplankton and bacteria in the field is more difficult (for example, refs 8 , 23 , 69 ). Testing upsurge hypothesis We tested whether biomass of fish (g per individual), zooplankton (g m −2 sediment) and bacteria (numbers per l), increased with the amount of OM in the first trophic level below them in the lake food web using generalized linear models built from a priori hypotheses of underlying mechanisms (see Supplementary Materials ). We also modelled POC and DOC as functions of NDVI and POC, respectively. Our approach allowed us to test the relative importance of OM quality versus quantity in driving biomass stocks by incorporating FA composition of zooplankton (for fish), abundance of phytoplankton taxa and DOM structure measured using fluorescence spectroscopy (for zooplankton and bacteria), and different measures of wetland area (for POC and DOC). Where appropriate, we also accounted for variation in biomass estimates simply due to habitat quality, that is, water chemistry, temperature and predation pressure. Measurement of OM and habitat quality is described in Supplementary Methods . Testing site affinity of fish We verified that fish populations foraged in the sites in which they were captured using concentrations of trace metals. We measured Al, Ba, Ca, Cd, Cr, Cu, Fe, K, Mg, Mn, Na, Ni, Se, Sr and Zn in ten fish from each site with inductively coupled plasma mass spectrometry. Fish size significantly influenced 10 of the 15 total-body metal concentrations; thus, we first removed these effects by fitting models to predict metal concentrations m i in each fish i with weight f i using linear ( m i =β 19 +β 20 f i ), exponential [log( m i )=β 21 +β 22 f i ] and inverse ( m i =β 23 +β 24 / f i ) functions. We used the Akaike information criterion to select the most strongly supported model for each possible metal, that is, lowest Akaike information criterion, and subtracted the β f i term from the element concentrations to calculate detrended values. We then used linear discriminant analysis in R v.2.15 to test whether detrended total-body metal concentrations could classify fish into unique groups corresponding with their site of origin. We also tested whether the molar ratios of Ba:Ca and Sr:Ca in fish reflected the water of sites from which fish were collected using a linear model (see Supplementary Methods for details). Trace elements such as Ba and Sr are particularly useful as habitat tracers because they are accumulated in CaCO 3 of bony structures found within fish at levels proportional to their environmental availability [70] . Testing terrestrial resource use We estimated the contribution of allochthonous OM sources to YOY fish within each site using a Bayesian three-isotope mixing model. We fitted the exact same model as Solomon et al. [23] , but added a hierarchical structure to account for variation in resource use among sites. Briefly, the model estimates the proportion of terrestrial, benthic and littoral primary production used by fish from stable isotope data and published physiological parameters (see Supplementary Methods ). It has the added benefits of incorporating covariates of isotopic ratios, uncertainty in source isotope data, dietary enrichment of δ 2 H and trophic fractionation of δ 15 N into estimates of resource use. By incorporating covariates of isotopic ratios, it also allowed us to test whether allochthonous support of fish populations increased with the vegetation and wetland cover of each site. We used periphyton and zooplankton as the sources of benthic and littoral production, respectively, because each integrates variability in both bacterial and algal production from their position in the water column spanning up to several weeks [7] , [23] , [68] , [69] . R code for the model is provided as Supplementary Software 1 . Statistical analyses We fitted all our models within a hierarchical Bayesian framework using Markov chain Monte Carlo sampling by calling JAGS v.3.3 from R and tested for convergence using three different approaches (see Supplementary Methods ). We calculated posterior means and 95% CIs for all parameter estimates and did not reject the upsurge hypothesis if 95% CIs for slopes describing relationships between quantities of biomass in adjacent trophic levels were positive and did not overlap zero. Validation of isotopic mixing model A criticism of our stable isotope mixing model is that we have underestimated terrestrial support of fish φ T, j , because we have used zooplankton as an end member in the model and zooplankton themselves consist of terrestrially derived resources. We can account for this in our isotopic mixing model by re-writing φ L, j as the sum of all the littoral resource use by fish minus the proportion that consists of terrestrial resources: ,where φ Tzoo ,j is the proportion of terrestrial resources supporting zooplankton. Correspondingly, we can re-write φ T, j as the sum of terrestrial resource used by fish independent of the component derived from zooplankton plus . Critically, it makes no difference whether we estimate φ T, j and φ L, j directly or the functions described here, given known estimates of φ Tzoo, j , which would be derived from a separate model fitted to zooplankton. We show this by simulating 15 observations across each of 8 sites with known mixing concentrations. By fitting our mixture model to these data ( Supplementary equations 9–11 ), we can re-cover the underlying mixture concentrations, despite the littoral end member consisting of terrestrial resources. Simulation code is provided as Supplementary Software 2 . Our approach was to sample at random eight observations from each of three distributions, whose means and s.d. were defined from δ 13 C-values observed for each of our three end-member sources, corresponding with terrestrial, littoral and benthic resources. This generated a different δ 13 C-value for each of the three sources in each of the eight sites. We then mixed the sources identically across the eight observations so as to combine 30% terrestrial, 60% littoral and 10% benthic resources, but allowed for 20% of the littoral resources to consist of leaf litter. Thus, the final contributions used to calculate values in our focal mixture were terrestrial=30%+20% × 60%=42% and littoral=60%–20% × 60%=48%; benthic values were unchanged. We treated these 8 values as ‘site means’ and each mean was added to 15 observations that were randomly drawn from a zero-mean normal distribution with s.d. equal to that observed for δ 13 C across all fish in our study. Overall, we produced 8 site means with 15 individual observations in each site, directly analogous to our empirical data. We repeated this for δ 15 N and δ 2 H, respectively, adding to mixtures the mean trophic enrichment Δ tot observed in our study and mean contributions of dietary water accounting for different trophic levels of end members (as described for Supplementary Equation 11 ). We then estimated our mixture model ( Supplementary Equations 9–11 ) using the approaches described in the Supplementary Methods . The entire procedure was repeated for 99 different simulated data sets, from which we calculated means and 95% CIs for φ coefficients. We successfully retrieved the final contributions of each end source to our mixture across the simulated data sets, negating any concern about underestimating terrestrial resource use. The mean (95% CI) of the terrestrial contribution was estimated to be 0.42 (0.37–0.47) across all our simulations, while the littoral contribution was 0.48 (0.42–0.54; Supplementary Fig. 7 ). These estimates closely matched the quantities used to derive the data of 0.42 and 0.48, respectively. Overall, the model was generally a good fit to the observed site mean (95% CI for R 2 : 0.74–0.96). How to cite this article: Tanentzap, A. J. et al. Forests fuel fish growth in freshwater deltas. Nat. Commun. 5:4077 doi: 10.1038/ncomms5077 (2014).